Reversible temperature regulation of electrical and thermal conductivity using liquid–solid phase transitions Reversible temperature tuning of electrical and thermal conductivities of materials is of interest for many applications, including seasonal regulation of building temperature, thermal storage and sensors. Here we introduce a general strategy to achieve large contrasts in electrical and thermal conductivities using first-order phase transitions in percolated composite materials. Internal stress generated during a phase transition modulates the electrical and thermal contact resistances, leading to large contrasts in the electrical and thermal conductivities at the phase transition temperature. With graphite/hexadecane suspensions, the electrical conductivity changes 2 orders of magnitude and the thermal conductivity varies up to 3.2 times near 18 °C. The generality of the approach is also demonstrated in other materials such as graphite/water and carbon nanotube/hexadecane suspensions. Reversible temperature tuning of electrical and thermal conductivities of materials is of interest for many applications, such as seasonal regulation of building temperatures, thermal storage, sensing and so on. Although the electrical conductivity can be tuned by temperature using metal-insulator transitions [1] , [2] , [3] , [4] , temperature regulation of thermal conductivity is much more difficult as thermal properties vary little through solid-state phase transitions. In particular, materials capable of near room temperature regulation of both electrical and thermal conductivity could prove useful for new applications. Liquid–solid phase transitions can be an attractive route for the temperature regulation of electrical and/or thermal properties because of the availability of materials with a wide range of phase transition temperatures. Because a liquid–solid phase transition usually does not cause a metal-insulator transition, nanoparticles can be added to liquids to control the property contrast between the liquid and solid states. In particular, in a crystal-forming liquid loaded with nanoparticles, particles are squeezed towards grain boundaries on freezing [5] , [6] , [7] . The internal stress generated during freezing regulates the contacts among particulates, increasing the electrical and/or thermal conductivities of the composites. The changes of the electrical and/or thermal conductivities at the phase transition temperature can be further optimized by adjusting the concentration of the particulates. By combining these effects, novel composites exhibiting large variations in electrical and thermal conductivities in a narrow room temperature range can be achieved. In this paper, we demonstrate this first-order phase-transition strategy to regulate electrical and thermal properties. Using a graphite/hexadecane suspension as an example, we achieve a 2-orders-of-magnitude change in the electrical conductivity and a three-fold change in the thermal conductivity around 18 °C. The generality of the approach is also demonstrated in other materials such as graphite/water and carbon nanotube/hexadecane suspensions. The critical temperature of such temperature-responsive composites can be readily adjusted for specific applications by selecting host fluids with the right phase transition temperature. Sample preparation We use a hexadecane/graphite suspension as an example. The phase transition temperature of hexadecane is around 18 °C, which is convenient for experimentation. Exfoliated graphite flakes have been widely utilized in composite materials because of their high in-plane strength and high electrical and thermal conductivities [8] . We followed a process of sulphuric acid intercalation, microwave expansion and ultrasonic dispersion to prepare graphite suspensions [9] , [10] , [11] . After these processes, natural graphite is exfoliated into graphite flakes, which are then mixed with hexadecane to form a stable suspension. 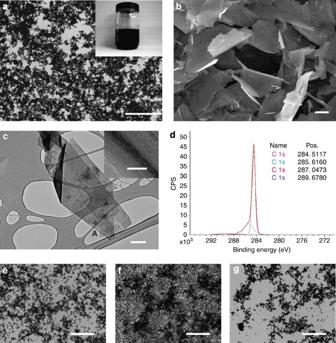Figure 1: Microstructures of graphite/hexadecane suspensions. (a) Optical microscope image of the microstructure of a 0.2% (volume fraction) graphite/hexadecane suspension; scale bar, 200 μm. The inset shows an optical photograph of a 50-ml, 0.2% graphite/hexadecane suspension after 3 months on the shelf. (b) A scanning electron micrograph of graphite flakes obtained by the H2SO4intercalation, microwave expansion and ultrasonic exfoliation of natural graphite; scale bar, 1 μm. (c) A typical transmission electron microscopy image of a graphite flake. The inset shows a high-resolution transmission electron microscopy image of the selected area (denoted by A). Scale bar incand inset correspond to 1 μm and 5 nm, respectively. (d) C1s X-ray photoelectron spectra of graphite flakes; the spectra have a main peak at 284.5 eV. The peak can be fit to peaks at 284.5, 285.6, 287.0 and 289.6 eV and thus assigned to theC=C,C−OH,C=OandO=C−OHspecies, respectively. (e) An optical microscope image of 0.05% graphite/hexadecane suspension. (f) An image of a frozen graphite/hexadecane composite. The black area represents graphite clusters, whereas the needle-like structure represents hexadecane grains. (g) The microstructure of a remelted graphite suspension showing the graphite percolation network. Scale bars ine,fandgare all corresponding to 200 μm. Suspension characteristics An optical microscope image of 0.2% (volume fraction) graphite/hexadecane suspension is shown in Figure 1a , together with an inset showing a photo of 50 ml of such a suspension after 3 months on the shelf. The graphite suspension is stable and no sediment is found. The graphite flakes have an average diameter of several microns and a thickness from several nanometres to several tens of nanometres ( Fig. 1b ). Because of the intrinsic stress induced during preparation, most of the graphite flakes are bent, with some of them even rolled up ( Fig. 1c ). A high-resolution transmission electron microscopy image (inset in Fig. 1c ) of a selected flake shows that the flake has ~30 atomic layers with an interplanar distance of 0.335 nm, consistent with graphite [7] . We measured the mobility of graphite flakes in hexadecane to be ~0.03 cm 2 V −1 s −1 , which means that the graphite flakes are charged in hexadecane. X-ray photon spectroscopy (XPS) analysis indicates that the surface of the graphite flakes contains ~8% oxygen atoms ( Fig. 1d ), which are contributed by the hydroxyl, epoxide and carboxyl groups on the graphite surface. These functional groups may have a significant role in the stability of the graphite suspensions [12] , [13] . Figure 1: Microstructures of graphite/hexadecane suspensions. ( a ) Optical microscope image of the microstructure of a 0.2% (volume fraction) graphite/hexadecane suspension; scale bar, 200 μm. The inset shows an optical photograph of a 50-ml, 0.2% graphite/hexadecane suspension after 3 months on the shelf. ( b ) A scanning electron micrograph of graphite flakes obtained by the H 2 SO 4 intercalation, microwave expansion and ultrasonic exfoliation of natural graphite; scale bar, 1 μm. ( c ) A typical transmission electron microscopy image of a graphite flake. The inset shows a high-resolution transmission electron microscopy image of the selected area (denoted by A). Scale bar in c and inset correspond to 1 μm and 5 nm, respectively. ( d ) C1s X-ray photoelectron spectra of graphite flakes; the spectra have a main peak at 284.5 eV. The peak can be fit to peaks at 284.5, 285.6, 287.0 and 289.6 eV and thus assigned to the C = C , C − OH , C = O and O =C− OH species, respectively. ( e ) An optical microscope image of 0.05% graphite/hexadecane suspension. ( f ) An image of a frozen graphite/hexadecane composite. The black area represents graphite clusters, whereas the needle-like structure represents hexadecane grains. ( g ) The microstructure of a remelted graphite suspension showing the graphite percolation network. Scale bars in e , f and g are all corresponding to 200 μm. Full size image The microstructure evolution of a dilute graphite/hexadecane suspension (0.05% graphite/hexadecane) during phase transition was imaged using an optical microscope. In the liquid phase, the graphite flakes attract each other forming graphite clusters ( Fig. 1e ). During freezing, the graphite flakes are pushed to the grain boundary by the anisotropic growth of needle-like hexadecane crystals, generating a three-dimensional percolation network ( Fig. 1f ). After the frozen hexadecane is remelted, the graphite percolation network persists while only a few isolated suspended graphite flakes could be observed ( Fig. 1g ). Freezing thus results in the local enhancement of the graphite concentration, which will further influence the transport properties of graphite suspensions. Electrical conductivity The electrical conductivity of the suspensions is measured using a four-point configuration. 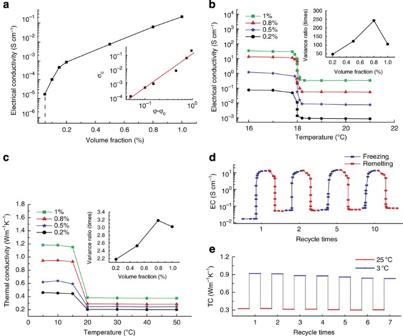Figure 2: Variation of electrical and thermal conductivities around the phase transition point. (a) Electrical conductivity of graphite suspensions as a function of volume fraction in the liquid state. The inset shows a logarithmic plot ofσcversus (ϕ−ϕc), which indicates a percolation threshold ofϕc=0.05%. (b) Electrical conductivity of graphite suspensions as a function of temperature. The inset shows the relationship between the contrast ratio of electrical conductivity and graphite volume fraction. (c) Thermal conductivity at different graphite volume fractions as a function of temperature. The inset plot indicates the relationship between the contrast ratio of thermal conductivity and graphite volume fraction. (d) Cyclic EC (electrical conductivity) versus temperature measurement results of a 0.8% graphite/hexadecane suspension. Blue and red squares indicate the conductivity variance through the processes of freezing and melting, respectively. (e) TC (thermal conductivity) contrast after different cycles. Blue lines indicate the thermal conductivity of 0.8% graphite/hexadecane suspensions at 3 °C during different thermal cycles, whereas red lines show the thermal conductivity at 25 °C during different thermal cycles. The electrical conductivities of the graphite suspensions in the liquid state prepared using different volume fractions of the graphite flakes are shown in Figure 2a . The inset of Figure 2a shows a logarithmic plot of electrical conductivity versus ( ϕ − ϕ c ), demonstrating a percolating threshold of ϕ c =0.05% (ref. 14 ). The electrical conductivity of the graphite suspensions varies significantly around 18 °C when hexadecane starts to freeze, as shown in Figure 2b for a graphite volume fraction loading between 0.2–1%, above the percolation threshold. In the liquid state, the electrical conductivity of the graphite suspensions varies little with temperature; from 18.5 to 17.5 °C, the electrical conductivity increases by 2 orders of magnitude. After the hexadecane is completely frozen, the electrical conductivity stabilizes. In both the solid and the liquid states, the electrical conductivity increases with an increase of the graphite volume fraction. However, the contrast ratio of electrical conductivity, defined as the ratio of electrical conductivity between the solid and the liquid states near the phase transition, peaks at 250 around a volume fraction of 0.8% ( Fig. 2b , inset). The peak exists because at a lower graphite volume fraction, the electrical conductivity in the solid state is not sufficiently high. However, at a higher graphite volume fraction, the electrical conductivity in the liquid state is large, also reducing the contrast ratio. We anticipate that the peak value depends on the geometry of the graphite flakes, surface states and liquid properties, and believe that further improvements in the contrast ratio are possible through optimization. Figure 2: Variation of electrical and thermal conductivities around the phase transition point. ( a ) Electrical conductivity of graphite suspensions as a function of volume fraction in the liquid state. The inset shows a logarithmic plot of σ c versus ( ϕ − ϕ c ), which indicates a percolation threshold of ϕ c =0.05%. ( b ) Electrical conductivity of graphite suspensions as a function of temperature. The inset shows the relationship between the contrast ratio of electrical conductivity and graphite volume fraction. ( c ) Thermal conductivity at different graphite volume fractions as a function of temperature. The inset plot indicates the relationship between the contrast ratio of thermal conductivity and graphite volume fraction. ( d ) Cyclic EC (electrical conductivity) versus temperature measurement results of a 0.8% graphite/hexadecane suspension. Blue and red squares indicate the conductivity variance through the processes of freezing and melting, respectively. ( e ) TC (thermal conductivity) contrast after different cycles. Blue lines indicate the thermal conductivity of 0.8% graphite/hexadecane suspensions at 3 °C during different thermal cycles, whereas red lines show the thermal conductivity at 25 °C during different thermal cycles. Full size image Thermal conductivity The thermal conductivity is measured using a hot-wire method [15] . The thermal conductivity of the graphite suspensions has the same trend as the electrical conductivity ( Fig. 2c ). In the liquid state, thermal conductivity changes little with temperature. As the host solidifies, the thermal conductivity rises sharply. At 0.8% volume fraction, it was observed that the thermal conductivity changes by a factor of 3.2 near the phase transition temperature ( Fig. 2c , inset). The smaller contrast in the thermal conductivity change compared with that of electrical conductivity is because of the fact that the thermal and electrical transport mechanisms are different. Electrons are forced to pass only through the graphite flakes, whereas heat can conduct through both the liquid and the solid host phases. Furthermore, the thermal conductivity ratio between graphite and hexadecane is ~10 4 , whereas for the electrical transport the ratio of conductivities can be on the order of 10 12 –10 16 . Reversibility The cycling behaviour of the electrical conductivities as the materials go through repeated melting and solidification processes is shown in Figure 2d . The first freezing cycle shows the largest contrast in electrical conductivities because there are more loose clusters in the liquid states. When the frozen hexadecane remelts, the contact between graphite flakes degrade quickly, leading to sharp reductions in the electrical conductivity. However, many graphite flakes will be trapped in the percolation network and the electrical conductivity in the liquid state increases from its original as-synthesized state. After the first temperature cycle, the percolation structure becomes stable, and thus the contrast ratio of the electrical conductivity of the suspension approaches a constant. All the experimental data shown in Figure 2b,c are the result of the second freezing cycle of different samples. The cycling behaviour of the thermal conductivity was shown in Figure 2e . The variation of thermal conductivity during the first and subsequent cycles is smaller because unlike electrical conductivity, heat conducts through both the graphite percolation network and the host. The experimental results presented in Figure 2b–e were obtained for suspensions that already reached percolation in the liquid state. Thus, the large contrasts observed in the electrical and thermal conductivity changes at the phase transition are not simply due to the percolation structure. The internal stress generated during freezing may be responsible for the large contrasts through regulation of the contact resistances of the percolated nanoparticle network. We set up an experiment ( Fig. 3a ) to measure the electrical contact resistance between two highly ordered pyrolytic graphite ( SPI-1 ) flakes in a hexadecane environment. The resistance of the circuit decreases 400 times as the temperature decreases from 18.5 to 17.5 °C ( Fig. 3b ). The stress distribution ( Fig. 3c ) measured in the frozen hexadecane (see Method) shows that the stress is unevenly distributed in regions where the average pressure is ~160 p.s.i. We believe the non-uniform pressure distribution is due to the anisotropic growth of hexadecane crystals. 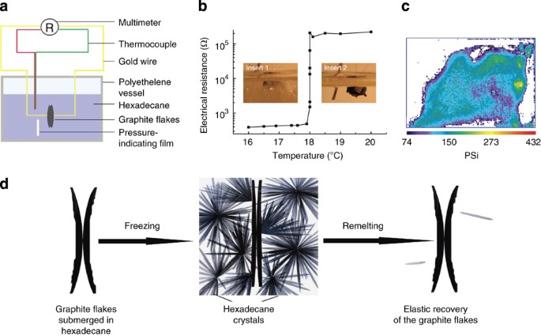Figure 3: Mechanisms in reversible temperature control of both electrical and thermal conductivities. (a) Schematic diagram of measurement of electrical resistance between two graphite flakes peeled from highly ordered pyrolytic graphite. The dimensions of the graphite flakes are ~1 μm×3 mm×3 mm. Graphite flakes are contacted by 30-μm diameter gold wires. (b) Measured variation of electrical resistance as a function of temperature, from 18.5 to 17.5 °C. The resistance of the circuit decreased about 460 times. Inset 1 is an optical image of graphite flakes submerged in solid hexadecane, and inset 2 shows the graphite flakes submerged in liquid hexadecane. (c) Stress distribution map in frozen hexadecane, showing that the stress is unevenly distributed from 74–400 p.s.i., with an average of ~160 p.s.i. (d) Conceptual illustration of the contact area variation between graphite flakes submerged in hexadecane through the process of hexadecane freezing and remelting. The anisotropic growth of hexadecane crystals generates pressure on the surface of the graphite flakes, which increases the contact area and reduces the flake separation. When the frozen hexadecane remelts, the pressure is released and the contact area decreases. The conceptual process is shown in Figure 3d . Similar to exfoliated graphite flakes, naturally peeled highly ordered pyrolytic graphite flakes are uneven and curved. In the liquid state, the contact area is small and hence the electrical resistance between two flakes is high. Hexadecane crystals exhibit strong anisotropic growth kinetics. During the freezing of hexadecane needle-like structures are formed, with the aspect ratio depending mainly on the freezing speed. The anisotropic growth of the hexadecane crystals generates stress and increases the contact area of the graphite flakes. Stress can also improve the electrical contacts by reducing the thickness of the insulating liquids in between graphite flakes. After freezing, the contact area and electrical resistance stabilize. When the hexadecane remelts, the pressure on the graphite flakes is released and the contact area is reduced because of the elastic recovery of the graphite flakes and interparticle repulsion. A similar trend exists for the thermal conductivity as well. Figure 3: Mechanisms in reversible temperature control of both electrical and thermal conductivities. ( a ) Schematic diagram of measurement of electrical resistance between two graphite flakes peeled from highly ordered pyrolytic graphite. The dimensions of the graphite flakes are ~1 μm×3 mm×3 mm. Graphite flakes are contacted by 30-μm diameter gold wires. ( b ) Measured variation of electrical resistance as a function of temperature, from 18.5 to 17.5 °C. The resistance of the circuit decreased about 460 times. Inset 1 is an optical image of graphite flakes submerged in solid hexadecane, and inset 2 shows the graphite flakes submerged in liquid hexadecane. ( c ) Stress distribution map in frozen hexadecane, showing that the stress is unevenly distributed from 74–400 p.s.i., with an average of ~160 p.s.i. ( d ) Conceptual illustration of the contact area variation between graphite flakes submerged in hexadecane through the process of hexadecane freezing and remelting. The anisotropic growth of hexadecane crystals generates pressure on the surface of the graphite flakes, which increases the contact area and reduces the flake separation. When the frozen hexadecane remelts, the pressure is released and the contact area decreases. Full size image The strategy demonstrated with a graphite-hexadecane suspension is general. Both the fluids and the particulates can be changed to optimize for specific applications. The base fluid should be a material that is crystalline in the solid state. The particulates could be any material with high electrical and/or thermal conductivity that can form a stable suspension when the host material is in the liquid state. 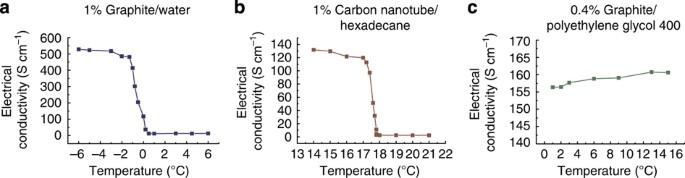Figure 4: The electrical conductivity of three other suspensions. (a) 1% graphite/water suspension. The electrical conductivity decreases about 24 times from −0.5 to 0.5 °C. (b) 1% carbon nanotube/hexadecane suspension. The electrical conductivity decreases about 40 times from 17.5 to 18.5 °C. (c) 0.4% graphite/polyethylene glycol 400 suspension. Polyethylene glycol 400 (Alfa Aesar) has a melting point between 4 and 8 °C and does not form a crystalline solid. Consequently, no large variation in the electrical resistivity was observed. Figure 4a ,b shows similar behaviour in the temperature-dependent electrical conductivity variation of graphite/water suspensions and carbon nanotube/hexadecane suspensions. Figure 4c presents experimental results on a non-crystalline-forming suspension, made from polyethylene glycol 400 and graphite flakes, which shows no sharp change in the electrical conductivity during phase transition, further confirming the importance of a crystalline forming liquid host. Figure 4: The electrical conductivity of three other suspensions. ( a ) 1% graphite/water suspension. The electrical conductivity decreases about 24 times from −0.5 to 0.5 °C. ( b ) 1% carbon nanotube/hexadecane suspension. The electrical conductivity decreases about 40 times from 17.5 to 18.5 °C. ( c ) 0.4% graphite/polyethylene glycol 400 suspension. Polyethylene glycol 400 (Alfa Aesar) has a melting point between 4 and 8 °C and does not form a crystalline solid. Consequently, no large variation in the electrical resistivity was observed. Full size image In summary, we have demonstrated an effective strategy to tune the electrical and thermal conductivities of materials, using first-order phase transitions between liquid and crystalline solid states through seeding the liquid with particulates to form stable suspensions. During the phase transition, internal stress reduces the electrical and thermal contact resistances in the percolated network formed by the particulates, leading to large changes in the electrical and/or thermal conductivities. The strategy is general and can be tailored for either electrical and/or thermal conductivity or both, and for operation in a desired temperature range. Reversible tuning of electrical and thermal properties near room temperature as demonstrated in this paper has potential applications in temperature regulation and sensing. Extension of the method, such as using high melting point materials, for example, molten salts and ionic liquids, can be applied to solar thermal energy storage and power generation. Temperature regulation of the properties of the materials through percolation networks and stress generation during crystallization as demonstrated in this paper complements other actively controlled suspensions such as magnetorheological fluids and ferrofluids [16] , [17] . Sample preparation Exfoliated graphite was prepared from natural graphite (Asbury Carbons) by a chemical intercalation and thermal expansion method. A volume of 85 ml of H 2 SO 4 (96%, Alfa Aesar) and 15 ml of hydrogen peroxide (30%, Alfa Aesar) were mixed to form an oxidative agent that was used for the intercalation. For the intercalation process, 2.2 g of natural graphite was reacted with 100 ml of the oxidative agent at room temperature for 60 min. The slurries were rinsed with distilled water (Mallinckrodt Baker) to remove residual salts and acids, followed by filtering and baking on a hotplate at 110 °C for 24 h. The expanded graphite was obtained by thermal expansion of as-prepared graphite intercalation compounds in a 1,100-W commercial microwave oven (SANYO) for 30 s. The expanded graphite was then dispersed in hexadecane and other liquids to create a 1% volume fraction of graphite suspension. Graphite flakes were directly exfoliated from expanded graphite by ultrasonication in hexadecane (Sigma-Aldrich) or distilled water, using a high-intensity ultrasonic probe (Sonics VC750 (Sonics), 750 W, 80% amplitude) for 15 min. The obtained uniform dispersion was then dispersed in hexadecane and other liquids and further ultrasonication was performed for 3 min to obtain 0.2, 0.4, 0.6 and 0.8% suspensions. The dispersions become stable suspensions after they cool to room temperature. Microstructure characterization The morphologies of expanded graphite and exfoliated graphite flakes were observed by s.e.m. (JEOL JSM-6320, JEOL). The microstructures of exfoliated graphite are examined using a transmission electron microscopy (JEOL 200cx, JEOL 2011, JEOL) at room temperature. The evolution of the clusters and percolating structures of the graphite flakes in hexadecane was observed by a Nikon multipurpose zoom microscope (AZ100). XPS samples were prepared by pressing graphite flakes into a 5-mm-diameter disc. The sample was analysed by using a Kratos AXIS Ultra Imaging X-ray Photoelectron Spectrometer. The data were processed by using the CasaXPS software. Electrical conductivity measurement The electrical resistance of graphite suspensions was measured by pouring graphite gels into a self-made conductivity cell that has two dipping parallel vertical copper electrodes ~4.85 cm apart and with an area of ~1.17 cm 2 . The resistances of the graphite suspensions varied from 1.2–10 MΩ. The parasitic resistance of the conductivity cell is ~0.8Ω, which is far below the sample resistance. The electrical conductivity of graphite gels is given by the equation σ = k / R , where R is the measured resistance and k =3.83 cm −1 is the cell constant. We estimate that the uncertainty in the electrical conductivity measurement is ~1.6%. Thermal conductivity measurement A transient hot-wire method [15] was used to measure the thermal conductivity of the graphite suspensions. A 50-μm diameter Pt wire with a 1.5-μm thick insulating adhesion layer was fully immersed in the samples. The wire was subjected to a current pulse of precisely known amplitude and the resulting temperature rise was determined as a function of time by monitoring changes in the electrical resistance of the wire. By analysing the temporal temperature profile using solutions to the heat conduction equation, we determined the thermal conductivity of each sample. Our analyses show that the uncertainty of our hot-wire thermal conductivity setup is ~1.1%, and can be mostly attributed to systematic uncertainty due to uncertainty in the hot-wire length. In addition, we participated in a round-robin to measure the thermal conductivity of nanofluids [18] , and our experimental results were within 2% of mean values. Internal stress measurement The internal stress distribution in hexadecane was measured by a pressure-indicating film (Pressurex from Sensor Products). A sealed 15×10 mm 2 Pressurex film was submerged in a hexadecane-filled cell. The cell was placed in an ice-water bath for an hour so that hexadecane solidifies. Further, the cell was exposed to the ambient temperature (22 °C) and the Pressurex film was removed after the hexdecane remelted. A greyscale stress distribution profile appeared on the Pressurex film, revealing the relative amount of pressure applied to the film due to solidification. Using the Topaq software (Sensor Products), the greyscale pressure distribution profile is rendered into a full-colour representation of the stress distribution. How to cite this article : Zheng, R. et al . Reversible temperature regulation of electrical and thermal conductivity using liquid–solid phase transitions. Nat. Commun. 2:289 doi: 10.1038/ncomms1288 (2011).